IL-7 signalling represses Bcl-6 and the TFHgene program The transcriptional repressor Bcl-6 is linked to the development of both CD4 + T follicular helper (T FH ) and central memory T (T CM ) cells. Here, we demonstrate that in response to decreased IL-2 signalling, T helper 1 (T H 1) cells upregulate Bcl-6 and co-initiate T FH - and T CM -like gene programs, including expression of the cytokine receptors IL-6Rα and IL-7R. Exposure of this potentially bi-potent cell population to IL-6 favours the T FH gene program, whereas IL-7 signalling represses T FH -associated genes including Bcl6 and Cxcr5 , but not the T CM -related genes Klf2 and Sell . Mechanistically, IL-7-dependent activation of STAT5 contributes to Bcl-6 repression. Importantly, antigen-specific IL-6Rα + IL-7R + CD4 + T cells emerge from the effector population at late time points post influenza infection. These data support a novel role for IL-7 in the repression of the T FH gene program and evoke a divergent regulatory mechanism by which post-effector T H 1 cells may contribute to long-term cell-mediated and humoral immunity. During the course of an immune response, CD4 + T helper cells identify invading pathogens, proliferate and secrete cytokines to aid in immune-mediated clearance of infection. This results in an initial expansion of effector CD4 + T cells. As pathogen is eliminated, the number of CD4 + T cells is reduced to avoid potential autoimmunity that may result from a prolonged effector T-cell response. During this contraction phase, long-lived CD4 + T cells—termed memory T cells—survive to respond more quickly and robustly should the immune system re-encounter the same pathogen. The development of comprehensive immunological memory requires the generation of cells that are capable of contributing to both long-term cell-mediated and humoral immune responses, and includes populations of both CD4 + central memory T (T CM ) and T-follicular helper (T FH ) cells. T CM cells are one of many CD4 + memory T-cell populations that also include effector memory (T EM ), resident memory (T RM ) and recirculating memory (T RCM ) cell types [1] , [2] , [3] . These diverse sets of memory cells have been primarily identified by their immune function, tissue location and cell surface receptor expression. Specifically, T CM cells are uniquely identified by the expression of the homing receptors L-selectin (CD62L, encoded by the gene Sell ) and Ccr7 (ref. 1 ). The expression of these two receptors allows for trafficking to the T-cell zones of secondary lymphoid areas where T CM cells can participate in cell-mediated immunity by engaging in antigen surveillance. T FH cells facilitate humoral immune responses by assisting B-lymphocytes with the production of pathogen-neutralizing antibodies [4] , [5] , [6] . T FH cells are defined in part by the expression of the cell surface receptor Cxcr5, which allows for homing to the B cell zones of secondary lymphoid organs [4] , [5] . Differentiation of the T FH cell subset is a complex and multi-step process. These steps include the initiation of the T FH gene program, denoted by an initial upregulation of a partial T FH -profile (that is, Bcl-6 and Cxcr5 expression), followed by a second stage, whereby full commitment to the germinal center T FH cell state occurs upon B-cell interaction and enhanced ICOS signalling [7] . Given the inherent complexity of this process, many questions remain regarding the genesis of T FH cell populations. For example, while T FH cells can and do develop during the initial response to antigen, it has also been demonstrated that other effector T-helper cell subsets are capable of adopting a T FH -like profile, making a ‘post-effector’ developmental pathway plausible as well [8] , [9] , [10] , [11] , [12] , [13] . These previous studies are important as they support the possibility that, in addition to effector T FH cells, other T-helper populations may assist in long-term antibody-mediated immunity by co-opting certain aspects of the T FH -cell gene program. It has been previously demonstrated that the transcriptional repressor Bcl-6 is required for T FH development [14] , [15] , [16] . Bcl-6 directs T FH differentiation, at least in part, by antagonizing the expression of a second transcriptional repressor, Blimp-1, a known negative regulator of T FH cell differentiation [12] , [14] , [15] , [16] . Interestingly, upregulation of Bcl-6 has also been implicated in the differentiation of CD4 + effector T cells into memory cells, including the T CM subset [17] , [18] , [19] , [20] . However, it is currently unclear how this increase in Bcl-6 expression initiates this effector-to-memory transition. As with T FH differentiation, it has been postulated that a key function of Bcl-6 in promoting memory cell formation is to repress the expression of Blimp-1, a factor positively linked to the terminal differentiation of the effector cell state [2] , [21] , [22] , [23] . However, whether there are additional roles or long-term requirements for Bcl-6 expression in establishing T CM -cell fate apart from Blimp-1 repression remains unclear. Although transcription factors such as Bcl-6 are responsible for regulating the gene expression profiles of developing cells, upstream environmental signals, often in the form of a cytokine-dependent response, regulate the expression and/or the functional activity of individual transcription factors [24] . For example, it has been demonstrated that strong interleukin-2 (IL-2) signalling inhibits T FH formation by controlling the expression of Bcl-6 and Blimp-1 (refs 12 , 25 , 26 , 27 ). Similarly, it has been shown that inflammatory cytokine environments, including those that are IL-2 rich, can inhibit memory cell formation [28] , [29] . Collectively, evidence in the literature suggests that, despite their distinct functions and localization during the adaptive immune response, T FH and T CM cells share specific regulatory requirements and developmental programs. In addition, several recent studies have reported a high degree of similarity between T FH and T CM cells at the transcriptional and protein expression levels [9] , [17] , [19] , [30] . Furthermore, populations of memory T FH and T CM cells similarly express a number of cell surface receptors including Cxcr5, CD62L and Ccr7 (refs 8 , 9 , 30 , 31 , 32 ). Thus, there are precedents supporting the possibility that these two immune cell populations may be developmentally linked. However, as the contribution of each of these cells to long-term immunity is functionally distinct, it is likely that at some point there is a divergence to unique cytokine and transcriptional networks to allow for specialized T FH - and T CM -dependent immune responses. Here, we demonstrate that T-helper 1 (T H 1) cells are capable of co-initiating the expression of both T FH and T CM gene programs in response to decreased IL-2 signalling. Mechanistically, the initial co-expression of the T FH and T CM programs is due to the Bcl-6-dependent repression of Blimp-1. In addition, during this post-effector stage, T H 1 cells downregulate IL-2Rα expression, while upregulating the dual expression of IL-6Rα and IL-7R. This apparent cytokine receptor reprogramming results in a population of bi-potent ‘T FH /T CM -like’ cells with the ability to respond to either IL-6 or IL-7. Strikingly, while treatment with IL-6 results in the upregulation of Bcl-6 and Cxcr5 expression, exposure of these cells to IL-7 results in a dose-dependent decrease in T FH -associated genes including Bcl-6, while allowing the continued expression of T CM -specific genes. Importantly, at late time points post influenza infection, a population of antigen-specific IL-6Rα + IL-7R + CD4 + T cells emerges coincident with a decline in the effector population. Thus, this study describes a novel role for IL-7 in the repression of the T FH gene program and defines a potential mechanism by which post-effector T H 1 cells may be able to support aspects of both long-term cell-mediated and humoral immunity. IL-2 signalling modulates T H 1, T FH and T CM gene expression Our previous studies demonstrated that reduced IL-2 signalling has the potential to regulate T-helper cell fate decisions by augmenting the expression of the T FH lineage-defining factor Bcl-6 (ref. 12 ). In addition to its required role in T FH cell development, Bcl-6 expression has also been implicated in the formation of memory CD4 + T cells [1] , [17] , [19] , [20] . As such, we examined whether the IL-2-sensitive increase in Bcl-6 expression would similarly result in the upregulation of a memory cell gene program by exposing in vitro generated T H 1 cells to both high and low IL-2 concentrations. As with our prior study, the expression of a number of T H 1 genes was decreased in low environmental IL-2 conditions, while the expression of key T FH genes was induced, including the expression of Bcl6 and Cxcr5 ( Fig. 1a,b ). Consistent with the increase in transcript, Bcl-6 protein and cell surface expression of Cxcr5 were significantly increased ( Fig. 1c,d ). Interestingly, in addition to the induction of the T FH -like profile, T H 1 cells exposed to a low IL-2 concentration also upregulated genes associated with the T CM cell type—most notably the lymph node homing receptors Sell and Ccr7 ( Fig. 1e ) [1] , [2] , [33] . We also observed increased expression of other memory T-cell-related markers ( Il7r, S1pr1 , Cd27 and Cxcr3 ) and transcription factors known to promote the memory T-cell fate ( Klf2 , Klf3 and Foxo1 ; Fig. 1e,f ). Interestingly, the expression of Tcf7 , the gene that encodes the transcriptional regulator TCF-1, was significantly increased ( Fig. 1f ). Similar to Bcl-6, the expression of TCF-1 has been implicated in the development of both T FH and memory cells [34] , [35] , [36] , [37] , [38] . Importantly, the induction of the T CM -like profile was not limited to changes in transcript alone, as the cell surface expression of both CD62L and Ccr7 was significantly increased compared with that observed in effector T H 1 cells ( Fig. 1g,h ). Collectively, these data demonstrate that increased Bcl-6 expression in T H 1 cells, in response to decreased IL-2 signalling, results in the induction of not only a T FH -like profile, but a T CM -like profile as well. Furthermore, these data suggest that a common Bcl-6-dependent regulatory mechanism may be responsible for the initiation of both the T FH and T CM gene programs. 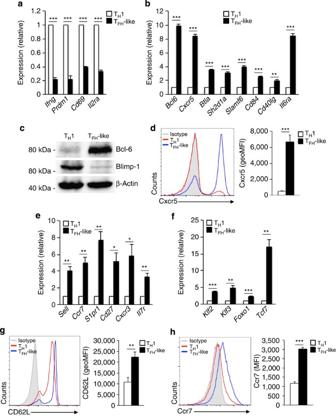Figure 1: IL-2 signalling regulates Bcl-6 expression in post-effector TH1 cells to allow for the upregulation of TFH- and TCM-like profiles. Primary CD4+T cells were cultured in TH1 conditions and exposed to either high (TH1 cells) or low (TFH-like cells) environmental IL-2 (250 U ml−1or 10 U ml−1, respectively). (a,b) RNA was isolated from the TH1 (white bar) and TFH-like (black bar) cells and the expression of the indicated genes was determined by quantitative RT–PCR. Data were normalized toRps18as a control and the results are represented as fold change in expression relative to the TH1 sample (mean ofn=3±s.e.m.). (c) An immunoblot analysis was performed to assess changes in protein expression in response to alterations of environmental IL-2. Expression for Bcl-6 and Blimp-1 was measured with β-actin serving as a control for equal protein loading. Shown is a representative blot of three independent experiments performed. (d) Representative histogram overlay of cell surface expression of Cxcr5 for TH1 and TFH-like cells. Geometric mean fluorescence intensity (geoMFI) for Cxcr5 is also shown (mean ofn=5±s.e.m.). (e,f) qRT–PCR analysis examining expression of the indicated genes in TH1 and TFH-like cells. Data were normalized and represented as inaandb(mean ofn=3±s.e.m.). (g,h) Representative histogram overlay of cell surface expression of (g) CD62L and (h) Ccr7 for TH1 and TFH-like cells. Average geoMFI or MFI for CD62L and Ccr7 expression are shown (mean ofn=5 or 4±s.e.m.). *P<0.05, **P<0.01, ***P<0.001 (unpaired Student’st-test). Figure 1: IL-2 signalling regulates Bcl-6 expression in post-effector T H 1 cells to allow for the upregulation of T FH - and T CM -like profiles. Primary CD4 + T cells were cultured in T H 1 conditions and exposed to either high (T H 1 cells) or low (T FH -like cells) environmental IL-2 (250 U ml −1 or 10 U ml −1 , respectively). ( a , b ) RNA was isolated from the T H 1 (white bar) and T FH -like (black bar) cells and the expression of the indicated genes was determined by quantitative RT–PCR. Data were normalized to Rps18 as a control and the results are represented as fold change in expression relative to the T H 1 sample (mean of n =3±s.e.m.). ( c ) An immunoblot analysis was performed to assess changes in protein expression in response to alterations of environmental IL-2. Expression for Bcl-6 and Blimp-1 was measured with β-actin serving as a control for equal protein loading. Shown is a representative blot of three independent experiments performed. ( d ) Representative histogram overlay of cell surface expression of Cxcr5 for T H 1 and T FH -like cells. Geometric mean fluorescence intensity (geoMFI) for Cxcr5 is also shown (mean of n =5±s.e.m.). ( e , f ) qRT–PCR analysis examining expression of the indicated genes in T H 1 and T FH -like cells. Data were normalized and represented as in a and b (mean of n =3±s.e.m.). ( g , h ) Representative histogram overlay of cell surface expression of ( g ) CD62L and ( h ) Ccr7 for T H 1 and T FH -like cells. Average geoMFI or MFI for CD62L and Ccr7 expression are shown (mean of n =5 or 4±s.e.m.). * P <0.05, ** P <0.01, *** P <0.001 (unpaired Student’s t -test). Full size image Blimp-1 inhibits the T CM -associated genes Sell and Ccr7 We previously identified Blimp-1 as a factor responsible for directly repressing members of the T FH gene program including Cxcr5 and Il6ra [12] . A key finding from our prior studies was that in response to reduced IL-2 signalling, Bcl-6 expression increased in T H 1 cells, resulting in the Bcl-6-dependent repression of Blimp-1 and the subsequent induction of the T FH gene program ( Fig. 1c ) [12] , [39] . Given our finding that increased Bcl-6 expression also leads to the induction of a T CM -like profile, we hypothesized that the same mechanistic interplay between Bcl-6 and Blimp-1 that results in the promotion of the T FH program may also initiate the transition from an effector T H 1 to a T CM -like cell state. Therefore, we examined whether T CM genes, similar to T FH genes, were direct Blimp-1 targets in effector T H 1 cells. Using predictive transcription factor binding site software (Genomatix), we identified potentially functional Blimp-1 DNA-binding elements in the promoters of both Sell and Ccr7 . To determine whether the predicted elements were functional, we prepared promoter–reporter constructs encompassing the predicted sites and performed luciferase reporter experiments in the presence and absence of overexpressed Blimp-1. Importantly, the expression of Blimp-1 resulted in a decrease in the promoter activity of both Sell and Ccr7 ( Fig. 2a,b ). As a control, there was no Blimp-1-mediated repression of a Tbx21 -reporter, which lacks predicted Blimp-1 DNA-binding elements. To determine whether Blimp-1-mediated repression may be the result of direct DNA binding, we performed promoter–reporter experiments with a mutant Blimp-1 construct lacking the zinc finger DNA-binding domain (ΔZF). Although wild-type Blimp-1 readily repressed promoter activity, there was no repression with the Blimp-1ΔZF protein ( Fig. 2c,d ). As a further test of the functional nature of the predicted sites, a Sell -reporter construct lacking the Blimp-1 DNA-binding element (pGL3- Sell ΔBL1) was not repressed by Blimp-1 ( Fig. 2e,f ). 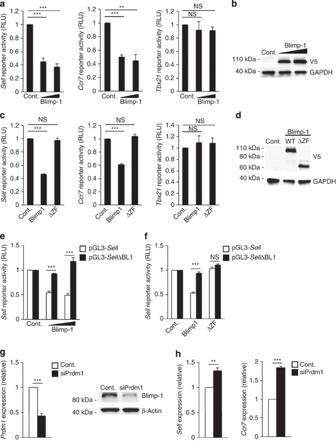Figure 2: Blimp-1 represses the CD4+TCMgenesSellandCcr7. (a,c,e,f) EL4 T cells were transfected with the indicated promoter–reporter constructs in combination with a wild-type Blimp-1 expression vector, a Blimp-1 mutant incapable of binding to DNA (ΔZF), or an empty vector control (mean ofn=3±s.e.m.). Ineandf, EL4 T cells were transfected with either a wild-typeSellpromoter–reporter or aSellpromoter–reporter lacking the predicted Blimp-1 DNA-binding elements (pGL3-SellΔBL1). Luciferase promoter–reporter values were normalized to arenillacontrol and expressed relative to the control sample for each experiment (mean ofn=4±s.e.m.). (b,d) Wild-type and mutant Blimp-1 protein levels were measured by immunoblot analysis. Shown is a representative blot of three independent experiments performed. (g,h) TH1 cells were nucleofected with either siRNA specific to Blimp-1 (siPrdm1) or a control siRNA. Following a 24-h time period, RNA was harvested and expression ofSellorCcr7was assessed by qRT–PCR. The data are presented as fold change in expression relative to the control sample (mean ofn=4±s.e.m.). **P<0.01, ***P<0.001 (unpaired Student’st-test). Cont., control; NS, not significant; WT, wild type. Figure 2: Blimp-1 represses the CD4 + T CM genes Sell and Ccr7 . ( a , c , e , f ) EL4 T cells were transfected with the indicated promoter–reporter constructs in combination with a wild-type Blimp-1 expression vector, a Blimp-1 mutant incapable of binding to DNA (ΔZF), or an empty vector control (mean of n =3±s.e.m.). In e and f , EL4 T cells were transfected with either a wild-type Sell promoter–reporter or a Sell promoter–reporter lacking the predicted Blimp-1 DNA-binding elements (pGL3- Sell ΔBL1). Luciferase promoter–reporter values were normalized to a renilla control and expressed relative to the control sample for each experiment (mean of n =4±s.e.m.). ( b , d ) Wild-type and mutant Blimp-1 protein levels were measured by immunoblot analysis. Shown is a representative blot of three independent experiments performed. ( g , h ) T H 1 cells were nucleofected with either siRNA specific to Blimp-1 (siPrdm1) or a control siRNA. Following a 24-h time period, RNA was harvested and expression of Sell or Ccr7 was assessed by qRT–PCR. The data are presented as fold change in expression relative to the control sample (mean of n =4±s.e.m.). ** P <0.01, *** P <0.001 (unpaired Student’s t -test). Cont., control; NS, not significant; WT, wild type. Full size image To examine the extent of Blimp-1-specific repression in an endogenous setting, we utilized a knockdown approach to assess the effect of decreasing Blimp-1 levels on the expression of these genes in effector T H 1 cells ( Fig. 2g ). Upon small interfering RNA (siRNA) knockdown of Blimp-1 expression, we observed a modest but significant increase in both Sell and Ccr7 expression ( Fig. 2h ). Collectively, these data suggest that the T CM -associated genes Sell and Ccr7 are repressed by Blimp-1 in effector T H 1 cells. Furthermore, these findings suggest that the repression of Blimp-1 by Bcl-6 is a critical event for the initiation of both T FH and T CM gene programs in T H 1 cells. T H 1 cells undergo cytokine receptor reprogramming T CM and T FH cell differentiation represent complex- and multistep processes that are directed by a litany of factors. A key determinant that influences immune cell differentiation is the cytokine environment to which the cell is exposed, as well as the ability of that cell to sense and respond to its environment through cytokine receptor expression. Our data indicate that effector T H 1 cells upregulate both T CM - and T FH -like gene expression patterns in response to a low IL-2 environment. Importantly, IL-2-signalling is known to influence the expression of cytokine receptors [40] . Initially, Il2ra is expressed at high levels in the effector T H 1 cells. However, as these cells transition to a low IL-2 environment, our data demonstrate that Il2ra expression decreases, whereas the expression of Il6ra and Il7r increases ( Fig. 1a,b,e ). Hence, the predominant cytokine receptor expression pattern changes from one supportive of effector T H 1 cells, which are responsive to elevated IL-2, to one enriched with IL-6Rα and IL-7R—receptors that respond to cytokines favouring T FH and T CM development, respectively [41] , [42] , [43] , [44] , [45] , [46] . Furthermore, these data are suggestive of the intriguing possibility that three divergent cell types may emerge from the effector T H 1 population: a pre-T FH -like population (IL-6Rα + IL-7R − ), a pre-T CM -like population (IL-6Rα − IL-7R + ) and/or a bi-potent pre-T FH /T CM (IL-6Rα + IL-7R + ) population that may be capable of transitioning into either cell type. To address the above possibilities, we assessed the composition of both the high IL-2 and low IL-2- treated T H 1 populations by examining the cell surface expression of IL-6Rα and IL-7R. Consistent with our transcript analysis, the expression of both IL-6Rα and IL-7R was significantly upregulated, whereas IL-2Rα was downregulated, on the surface of the low IL-2-treated cells ( Fig. 3a–c ). Importantly, the majority of the low IL-2-treated cells displayed dual expression of these receptors (double positive ‘DP’, IL-6Rα + IL-7R + ), whereas comparably few of the DP cells were observed in the high IL-2-treated (T H 1) population ( Fig. 3d,e ). 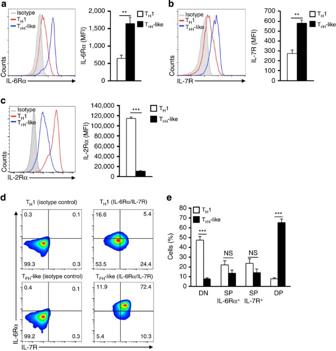Figure 3: TH1 cells undergo cytokine receptor reprogramming to dually express IL-6Rα and IL-7R. Primary CD4+T cells were cultured in TH1 conditions and exposed to either high (TH1 cells) or low (TFH-like cells) environmental IL-2 (250 U ml−1or 10 U ml−1, respectively). (a–e) Cell surface expression of IL-6Rα, IL-7R or IL-2Rα was measured by flow cytometric analysis. Data are represented as histograms (a–c), flow cytometry dot plots (d) or quantified percent positive cells (e). Average mean fluorescence intensity (MFI) for IL-6Rα, IL-7R and IL-2Rα expression is shown (mean ofn=3±s.e.m.). **P<0.01, ***P<0.001 (unpaired Student’st-test). DN, double negative; NS, not significant; SP, single positive. Figure 3: T H 1 cells undergo cytokine receptor reprogramming to dually express IL-6Rα and IL-7R. Primary CD4 + T cells were cultured in T H 1 conditions and exposed to either high (T H 1 cells) or low (T FH -like cells) environmental IL-2 (250 U ml −1 or 10 U ml −1 , respectively). ( a – e ) Cell surface expression of IL-6Rα, IL-7R or IL-2Rα was measured by flow cytometric analysis. Data are represented as histograms ( a – c ), flow cytometry dot plots ( d ) or quantified percent positive cells ( e ). Average mean fluorescence intensity (MFI) for IL-6Rα, IL-7R and IL-2Rα expression is shown (mean of n =3±s.e.m.). ** P <0.01, *** P <0.001 (unpaired Student’s t -test). DN, double negative; NS, not significant; SP, single positive. Full size image To confirm that the IL-6Rα + IL-7R + cells expressed both T FH -like and T CM -like programs, we sorted the DP population and compared the expression of key T H 1, T FH and T CM genes to that observed in effector high IL-2-treated (T H 1) and bulk low IL-2-treated (T FH -like) cells. Indeed, while significant differences were observed between the IL-6Rα + IL-7R + DP and effector T H 1 cells, the gene expression programs between sorted DP and bulk T FH -like cells were relatively indistinguishable ( Fig. 4 ). Consistent with the transcript analysis, IL-6Rα + IL-7R + cells also displayed elevated cell surface expression of CD62L, Ccr7 and Cxcr5 ( Supplementary Fig. 1a–c ). Collectively, these data support a model whereby, in response to reduced IL-2 signalling, T H 1 cells co-initiate the expression of both T FH and T CM -like gene programs, including the dual expression of IL-6Rα and IL-7R (hereafter referred to as ‘T FH /T CM -like’ cells). 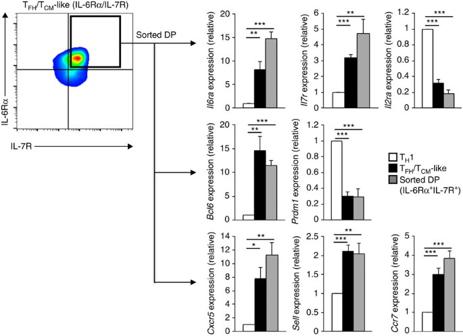Figure 4: Sorted IL-6Rα+IL-7R+double-positive (DP) cells dually express TFH- and TCM-like gene programs. Droplet digital PCR analysis was used to examine expression of TH1-, TFH- and TCM-associated genes. IL-6Rα+IL-7R+double-positive cells were sorted and their expression profiles were compared with that of TH1 (High IL-2) and TFH/TCM-like (Low IL-2) cells. Data were normalized toRps18and are represented as fold change in expression relative to the TH1 sample (mean ofn=4±s.e.m.). *P<0.05, **P<0.01, ***P<0.001 (unpaired Student’st-test). Figure 4: Sorted IL-6Rα + IL-7R + double-positive (DP) cells dually express T FH - and T CM -like gene programs. Droplet digital PCR analysis was used to examine expression of T H 1-, T FH - and T CM -associated genes. IL-6Rα + IL-7R + double-positive cells were sorted and their expression profiles were compared with that of T H 1 (High IL-2) and T FH /T CM -like (Low IL-2) cells. Data were normalized to Rps18 and are represented as fold change in expression relative to the T H 1 sample (mean of n =4±s.e.m.). * P <0.05, ** P <0.01, *** P <0.001 (unpaired Student’s t -test). Full size image IL-6 and IL-7 differentially regulate T FH and T CM genes The cytokines IL-6 and IL-7 have demonstrated roles in establishing and sustaining the T FH and T CM cell fates, respectively [41] , [42] , [43] , [44] , [45] , [46] . Therefore, to test the functional nature of IL-6Rα and IL-7R co-expression, we treated the T FH /T CM -like cells with either IL-6 or IL-7 and examined the expression of key T FH - and T CM -associated genes as compared with untreated controls. IL-6 treatment resulted in increased expression of the hallmark T FH genes Bcl6 and Cxcr5 , but did not significantly impact the expression of the T CM gene Sell ( Supplementary Fig. 2a,b ). Conversely, exposure to IL-7 resulted in a significant reduction in Bcl-6 expression and the repression of several other T FH genes ( Cxcr5 , Il6ra , Sh2d1a and Cd40lg ) ( Fig. 5a,b ). In many cases, the repression of the T FH -associated genes resulted in expression levels near to those observed in effector T H 1 cells. 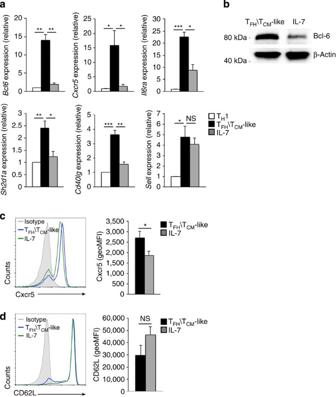Figure 5: IL-7 signalling represses Bcl-6 and TFHgene expression patterns. Primary CD4+T cells were cultured in TH1 conditions and exposed to either high or low environmental IL-2 to generate effector TH1 or TFH/TCM-like (IL-6Rα+IL-7R+) cells, respectively. TFH/TCM-like cells were then exposed to IL-7. Following a 24 or 48 h incubation, expression of the indicated genes was measured by (a) qRT–PCR, (b) immunoblot or (c,d) flow cytometric analysis. Fora, the sample values are presented as fold change in expression relative to the TH1 sample for each independent experiment (mean ofn=3±s.e.m.). Forb, Bcl-6 protein was measured with β-actin serving as a loading control. Shown is a representative blot of three independent experiments performed. Forcandd, data are represented either as histogram flow cytometry plots or quantified geometric mean fluorescence intensity (geoMFI; mean ofn=5±s.e.m.). *P<0.05, **P<0.01, ***P<0.001 (unpaired Student’st-test). NS, not significant. Figure 5: IL-7 signalling represses Bcl-6 and T FH gene expression patterns. Primary CD4 + T cells were cultured in T H 1 conditions and exposed to either high or low environmental IL-2 to generate effector T H 1 or T FH /T CM -like (IL-6Rα + IL-7R + ) cells, respectively. T FH /T CM -like cells were then exposed to IL-7. Following a 24 or 48 h incubation, expression of the indicated genes was measured by ( a ) qRT–PCR, ( b ) immunoblot or ( c , d ) flow cytometric analysis. For a , the sample values are presented as fold change in expression relative to the T H 1 sample for each independent experiment (mean of n =3±s.e.m.). For b , Bcl-6 protein was measured with β-actin serving as a loading control. Shown is a representative blot of three independent experiments performed. For c and d , data are represented either as histogram flow cytometry plots or quantified geometric mean fluorescence intensity (geoMFI; mean of n =5±s.e.m.). * P <0.05, ** P <0.01, *** P <0.001 (unpaired Student’s t -test). NS, not significant. Full size image As IL-7 is present at low levels in secondary lymphoid tissues, we next exposed the T FH /T CM -like cells to a range of physiologically relevant IL-7 concentrations and analysed the expression of key T CM and T FH genes ( Supplementary Fig. 3 ) [46] . Strikingly, even at an extremely low concentration of environmental IL-7, hallmark T FH genes ( Bcl6 , Cxcr5 and Il6ra ) were preferentially repressed. In stark contrast, the expression of the T CM -associated genes Sell , Klf2 and Ccr7 was relatively unaffected by IL-7 treatment. Importantly, the expression of the anti-apoptotic gene, Bcl2 , and the gene encoding the glycerol channel aquaporin 9, Aqp9 , both of which are known to promote the long-term survival of memory cells, was induced in response to IL-7 ( Supplementary Fig. 3 ) [47] , [48] . To further examine IL-7-induced changes to T FH and T CM cell surface marker expression, we compared Cxcr5 and CD62L protein expression in untreated T FH /T CM -like cells to those exposed to IL-7. Consistent with our transcript data, IL-7 treatment resulted in a significant reduction in Cxcr5 cell surface expression ( Fig. 5c ). In contrast, exposure to IL-7 resulted in a modest increase in CD62L, again suggesting that the repressive effect of IL-7 is limited to the T FH profile ( Fig. 5d ). It is important to note that in spite of the observed decrease in Cxcr5 expression, a majority of the Cxcr5 expressed on the cell surface remained refractory to the IL-7 repressive effect. This was in contrast to the almost complete loss of Bcl-6 protein expression in response to IL-7 treatment. These data corroborate other studies demonstrating that Cxcr5 expression can occur independent of Bcl-6 expression [13] , [49] . Furthermore, these data are consistent with the moderate expression of Cxcr5 observed on T CM cells [1] , [19] , [50] . IL-7-induced repression of Bcl-6 is independent of Blimp-1 The finding that IL-7 represses Bcl-6 expression has potentially far-reaching implications given the demonstrated roles for Bcl-6 in T FH development, T CM differentiation and in the regulation of cellular functions including metabolism and cell cycle progression [14] , [15] , [16] , [20] , [39] , [51] , [52] . As such, we sought to determine the identity of the transcription factor(s) responsible for directing IL-7-mediated repression of Bcl-6. There is a well-established inverse relationship between the transcriptional repressors Bcl-6 and Blimp-1 (refs 12 , 14 , 17 , 53 ). As our data demonstrate that IL-7-signalling inhibits Bcl-6 expression, we considered the possibility that IL-7 treatment may lead to increased Blimp-1 expression. To test this possibility, we examined the level of Prdm1 (Blimp-1) expression in T H 1 cells compared with that of T FH /T CM -like cells, and T FH /T CM -like cells exposed to IL-7 ( Fig. 6a ). Consistent with our previous results, T H 1 cells displayed significantly elevated expression of Prdm1 transcript as compared with T FH /T CM -like cells [12] . Interestingly, despite increased activation of STAT5 (which has been positively linked to Blimp-1 expression in response to IL-2 signalling), no appreciable increase in Blimp-1 protein was observed in the T FH /T CM -like cells stimulated with IL-7 ( Fig. 6b ). These data indicate that Blimp-1 is unlikely to be the IL-7-responsive factor that represses Bcl-6 expression. Furthermore, these data suggest that the IL-7-treated T FH /T CM -like cells are not simply reverting to a short-lived effector T H 1 phenotype (that is, possessing high Blimp-1 expression). Rather, it appears they are transitioning into cells with a gene program that more closely resembles that of long-lived T CM cells. 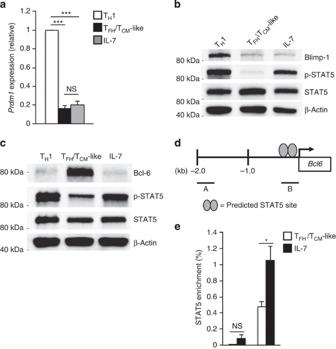Figure 6: IL-7-induced repression of Bcl-6 is mediated via STAT5 and independent of Blimp-1. (a) qRT–PCR or (b) immunoblot analysis of Blimp-1 expression in TH1, TFH/TCM-like cells, and TFH/TCM-like cells exposed to IL-7. Ina, data were normalized toRps18as a control and the results are presented relative to the TH1 sample (mean ofn=4±s.e.m.). Inb, protein expression was assessed using the indicated antibody. β-Actin was monitored as a control for equal protein loading. Shown is a representative blot of three independent experiments. (c) Immunoblot analysis of Bcl-6, phospho-STAT5 (p-STAT5) and STAT5 expression in primary TH1 cells, TFH/TCM-like cells and TFH/TCM-like cells exposed to IL-7. β-Actin was monitored to ensure equal protein loading. Shown is a representative blot of three independent experiments. (d) A schematic indicating the location of a predicted tetrameric STAT5 binding site in the promoter of theBcl6locus. PCR amplicons used in the chromatin immunoprecipitation (ChIP) analysis are indicated as ‘A’ and ‘B’. (e) ChIP assay to assess STAT5 association with theBcl6locus in response to IL-7-signalling. Data are represented as percent enrichment relative to a ‘total’ input sample (mean ofn=3±s.e.m.). *P<0.05, ***P<0.001 (unpaired Student’st-test). NS, not significant. Figure 6: IL-7-induced repression of Bcl-6 is mediated via STAT5 and independent of Blimp-1. ( a ) qRT–PCR or ( b ) immunoblot analysis of Blimp-1 expression in T H 1, T FH /T CM -like cells, and T FH /T CM -like cells exposed to IL-7. In a , data were normalized to Rps18 as a control and the results are presented relative to the T H 1 sample (mean of n =4±s.e.m.). In b , protein expression was assessed using the indicated antibody. β-Actin was monitored as a control for equal protein loading. Shown is a representative blot of three independent experiments. ( c ) Immunoblot analysis of Bcl-6, phospho-STAT5 (p-STAT5) and STAT5 expression in primary T H 1 cells, T FH /T CM -like cells and T FH /T CM -like cells exposed to IL-7. β-Actin was monitored to ensure equal protein loading. Shown is a representative blot of three independent experiments. ( d ) A schematic indicating the location of a predicted tetrameric STAT5 binding site in the promoter of the Bcl6 locus. PCR amplicons used in the chromatin immunoprecipitation (ChIP) analysis are indicated as ‘A’ and ‘B’. ( e ) ChIP assay to assess STAT5 association with the Bcl6 locus in response to IL-7-signalling. Data are represented as percent enrichment relative to a ‘total’ input sample (mean of n =3±s.e.m.). * P <0.05, *** P <0.001 (unpaired Student’s t -test). NS, not significant. Full size image IL-7 regulates STAT5 association with the Bcl6 promoter It is well established that the transcription factor STAT5 is activated downstream of IL-7 signalling [46] , [54] , [55] . Although STAT5 is known to function as a transcriptional activator, recent studies have described novel roles for STAT5 in the direct repression of gene expression [12] , [56] . To determine whether IL-7-signalling represses Bcl-6 expression through the activation of STAT5, we compared the activation state of STAT5 (p-STAT5) in effector T H 1, T FH /T CM -like cells and T FH /T CM -like cells exposed to IL-7 ( Fig. 6c ). Cells treated with IL-7 displayed elevated levels of STAT5 phosphorylation similar to that observed in effector T H 1 cells. In contrast, T FH /T CM -like cells had relatively low STAT5 activation. Importantly, the increased level of STAT5 activation in IL-7-treated cells correlated with decreased Bcl-6 expression. Given the inverse relationship between activated STAT5 and Bcl-6 expression, we hypothesized that STAT5 could play a role in the IL-7-mediated repression of Bcl-6 by directly binding to and repressing the Bcl6 promoter. In support of this hypothesis, a recent report demonstrated that a DNA sequence-specific tetrameric STAT5 complex functions downstream of IL-7R-signalling to repress gene expression during B-cell differentiation [56] . We analysed the Bcl6 locus and identified a potential tetrameric STAT5 DNA-binding site in the promoter region ( Fig. 6d ). We then performed chromatin immunoprecipitation (ChIP) analyses to determine whether STAT5 associates with the Bcl6 promoter in response to IL-7. Indeed, we detected increased STAT5 binding at the Bcl6 locus in T FH /T CM -like cells exposed to IL-7 as compared with untreated T FH /T CM -like cells ( Fig. 6e ). Importantly, the highest levels of STAT5 association corresponded to the location of the predicted tetrameric STAT5 binding site ( Fig. 6d,e ). Collectively, these data support a role for IL-7-activated STAT5 in the direct repression of Bcl-6 expression. IL-6Rα + IL-7R + CD4 + T cells emerge post influenza infection A key discovery from our in vitro experiments was that effector T H 1 cells upregulate both T FH and T CM gene programs in response to withdrawal of IL-2. These conditions are consistent with the late stages of an immune response, as the pro-inflammatory cytokine environment wanes and the effector population transitions to a memory population capable of supporting both cell-mediated and humoral immunity. Intriguingly, we observed that effector T H 1 cells undergo a period of cytokine receptor reprogramming in which they downregulate IL-2Rα, upregulate IL-6Rα and IL-7R, and initiate the expression of hallmark T FH and T CM genes. Therefore, to assess the kinetics of IL-6Rα and IL-7R expression in vivo , we infected mice with influenza (A/PR8/34; ‘PR8’) and monitored antigen-specific (nucleoprotein, ‘NP’-specific) CD4 + T cells at multiple time points post infection (days post infection, d.p.i.). Shortly after infection (9 d.p.i. ), cells could be divided into roughly two populations: effector T FH (Bcl-6 HI Cxcr5 HI ) and effector non-T FH (Bcl-6 MID Cxcr5 MID ). At this time point, the majority of the non-T FH effector population expressed low levels of IL-7R. However, at later time points (30 and 60 d.p.i. ), a substantial percentage of this population displayed increased expression of IL-7R ( Fig. 7a ). In comparison, T FH cells expressed relatively low levels of IL-7R, especially at late time points post infection ( Supplementary Fig. 4 ). Strikingly, the same cells that displayed increased expression of IL-7R also expressed the highest levels of IL-6Rα ( Fig. 7b ). Importantly, the IL-6Rα + IL-7R + DP population increased with time post infection, whereas effector T FH and non-T FH (IL-7R LO ) populations decreased ( Fig. 7c ). Collectively, these data indicate that a population of long-lived (60 d.p.i. ), antigen-specific IL6Rα + IL7R + DP cells arises during the post-influenza-infection period. Furthermore, the dual expression of IL-6Rα and IL-7R, in addition to our in vitro data demonstrating the differential regulation of T FH and T CM gene programs by IL-6 and IL-7, suggest that the activation of these cytokine-signalling pathways will likely influence the functional capabilities of the IL-6Rα + IL-7R + cells in vivo . 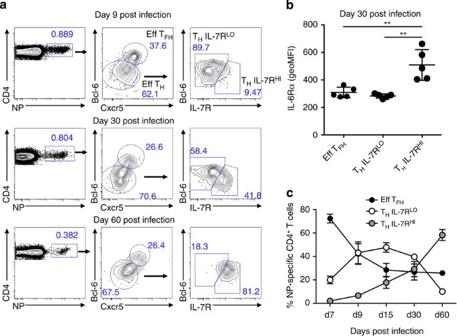Figure 7: IL-6Rα+IL-7R+CD4+T cells are detected at late time points post influenza infection. Mice were infected with influenza (PR8) and CD4+CD19−Foxp3−cells were analysed by flow cytometric analysis at the indicated day post infection. (a) Nucleoprotein (NP)-specific cells were isolated and sorted into effector TFH(Eff TFH) and non-TFH(Eff TH) populations. Non-TFHeffector cells were then assessed for IL-7R expression and further classified as IL-7R low (IL-7RLO) or IL-7R high (IL-7RHI). (b) IL-6Rα expression of the indicated cell population was measured by flow cytometric analysis (geometric mean fluorescence intensity (geoMFI); mean ofn=5±s.d.). (c) Percent NP-specific distribution of Eff TFH, THIL-7RLOand THIL-7RHIcells at the indicated time points (Day 7, d9, d15, d30, d60) post influenza infection (mean ofn=5±s.d.). **P<0.01 (unpaired Student’st-test). Figure 7: IL-6Rα + IL-7R + CD4 + T cells are detected at late time points post influenza infection. Mice were infected with influenza (PR8) and CD4 + CD19 − Foxp3 − cells were analysed by flow cytometric analysis at the indicated day post infection. ( a ) Nucleoprotein (NP)-specific cells were isolated and sorted into effector T FH (Eff T FH ) and non-T FH (Eff T H ) populations. Non-T FH effector cells were then assessed for IL-7R expression and further classified as IL-7R low (IL-7R LO ) or IL-7R high (IL-7R HI ). ( b ) IL-6Rα expression of the indicated cell population was measured by flow cytometric analysis (geometric mean fluorescence intensity (geoMFI); mean of n =5±s.d.). ( c ) Percent NP-specific distribution of Eff T FH , T H IL-7R LO and T H IL-7R HI cells at the indicated time points (Day 7, d9, d15, d30, d60) post influenza infection (mean of n =5±s.d.). ** P <0.01 (unpaired Student’s t -test). Full size image Following infection, the contraction of the effector response and the subsequent emergence of the memory cell population are vital to long-lasting immunity. However, the potential for memory populations to arise from the numerous CD4 + T-cell subsets, as well as the degree of plasticity that exists between these subsets, has complicated the identification of specific environmental signals and precise transcriptional networks that direct the effector-to-memory transition. For example, T FH and T CM cells appear to share developmental pathways, including requirements for the transcriptional repressor Bcl-6 and low levels of IL-2 signalling [14] , [15] , [16] , [19] , [20] . Interestingly, our data suggest that the T FH and T CM gene programs can co-initiate from a population of effector T H 1 cells upon increased Bcl-6 expression in response to IL-2 withdrawal, resulting in a ‘T FH /T CM -like’ population. In agreement with these data, there is emerging evidence for a set of genes which are linked to both T FH and memory cell development, including Bcl6 , Cxcr5 , Il7r and Tcf7 (refs 9 , 19 , 34 , 35 , 36 , 37 , 38 ). In addition, these data are physiologically intuitive as IL-2 signalling decreases during the late stages of an immune response, coincident with the formation of memory cell populations. Indeed, both T FH and T CM cells are required post contraction to mediate long-lasting humoral- and cell-mediated immunity, respectively. Therefore, it is likely that, following the initial co-expression of the T FH and T CM gene programs, there are distinct environmental and transcriptional regulatory mechanisms that promote T FH versus T CM -cell-dependent immune responses. In support of this divergence, we observed that T H 1 cells downregulate IL-2Rα while upregulating both IL-6Rα and IL-7R in response to a reduction in IL-2 signalling. Thus, these cells appear to reprogramme their ability to respond to both a T CM -essential (IL-7) and a T FH -associated (IL-6) cytokine. Our data further demonstrate that IL-6 treatment of T FH /T CM -like cells results in the further augmentation of the T FH profile. However, IL-7 exposure results in an inhibition of T FH genes, including Bcl-6. These findings highlight a previously unappreciated role for IL-7 in the repression of the T FH gene program in post-effector T H 1 cells. Importantly, they also suggest that Bcl-6 may only be required for the initiation of the T CM gene program, and that further developmental steps require a unique and undefined set of transcriptional regulators. Indeed, there are many reports in the literature describing a reduction in Bcl-6 expression in T CM cells at late time points post infection [7] , [13] , [19] , [30] , [57] . Furthermore, these findings are consistent with defined roles for Bcl-6 in the regulation of metabolism, cell cycle progression and apoptosis [39] , [46] , [47] , [51] , [52] , [58] , [59] . Thus, IL-7-dependent repression of Bcl-6 may ultimately be necessary to promote the unique sets of regulatory activities required for long-term memory cell survival. Interestingly, while IL-6 treatment augmented T FH gene expression, it did not affect the expression of T CM genes in the T FH /T CM -like post-effector population. Thus, these cells express hallmark genes of both T FH and T CM -cell types and resemble T FH -memory cells [50] . Whether there is a factor akin to IL-7 responsible for repressing the T CM -profile and promoting the T FH cell fate is a question that remains to be answered. In support of the model proposed here and perhaps shedding light on this question, recent reports have highlighted the antagonistic nature of T FH -associated ICOS signalling and the T CM transcription factor, Klf2. In these studies, ICOS signalling-dependent repression of Klf2 was required for commitment to the T FH -cell fate [60] , [61] . Thus, in addition to IL-6 signalling, interactions between T FH /T CM -like cells and B cells, along with the corresponding ICOS stimulation, are likely required to antagonize the T CM gene program and specifically promote T FH -dependent immune responses. Our data demonstrate that the IL-7-dependent repression of Bcl-6 is not a result of increased Blimp-1 expression. This is surprising, as these transcriptional repressors often appear in opposition during developmental steps in the immune system. Rather, our current data support a mechanism of transcriptional repression whereby activated STAT5 functions downstream of IL-7 signalling to repress Bcl-6 expression. This finding is similar to the inverse correlation between IL-2-dependent STAT5 activation and Bcl-6 expression that we reported in a prior study [12] . Interestingly, STAT5 has been shown to interact with the histone methyltransferase, Ezh2, downstream of IL-7 signalling [56] . As such, future experiments that determine whether there are cytokine-dependent differences to the composition of the STAT5 complex that binds to the Bcl6 locus could provide insight into how IL-7 and IL-2 harbour non-redundant roles in the regulation of immune cell development and function, despite signalling through a common downstream transcriptional regulator, STAT5 (refs 54 , 55 ). Collectively, this study supports a model in which effector T H 1 cells co-initiate T FH and T CM gene programs when IL-2 signals begin to wane. Our finding that antigen-specific effector CD4 + T cells upregulate the dual expression of IL-6Rα and IL-7R at late time points post influenza infection suggests that exposure to either cytokine could be a key determinant in further differentiation events and long-term cellular function. Although these findings may be indicative of divergence to either a T FH - or T CM -specific gene program, they do not preclude the possibility that plasticity exists between these cell states to influence trafficking between the T-cell and B-cell zones of secondary lymphoid tissues to provide a more comprehensive immune response. It is also possible that the simultaneous expression of IL-6Rα and IL-7R allow for precise modulation of Bcl-6 expression. A rheostatic model such as this may allow for modest Bcl-6 expression, sufficient to repress Blimp-1 expression and initiate the T CM transcriptional program, while also repressing the enhanced levels of Bcl-6 required for T FH development via IL-7 signalling. Future studies that address these possibilities by examining the functional properties of the IL-6Rα + IL-7R + CD4 + cells described here will be critical to enhance our understanding of the relationship between the T FH and T CM cell types. Primary cells and cell culture Primary naive CD4 + T cells were isolated from the spleen and lymph nodes of sex- and age-matched (5–8-week old) wild-type C57BL/6 mice using the MagCellect kit (R&D, MAGM205), consistently providing a 90–95% pure population. Following isolation, cells were cultured on plate-bound αCD3/αCD28 in T H 1 polarizing conditions (α-IL-4 (5 μg ml −1 ) and IL-12 (5 ng ml −1 )). After 3 days, cells were removed from αCD3/αCD28 stimulation, split and cultured for an additional 2 days in either high (250 U ml −1 ) or low IL-2 (10 U ml −1 ) conditions to generate effector T H 1 or T FH -like cells, respectively [12] . Low IL-2-treated cells were then treated with IL-6 (10 ng ml −1 ) or IL-7 (10 ng ml −1 ) unless otherwise indicated. Following a 24-h incubation, cells were collected for analysis. Primary T-cell transfections were performed with the 4D Lonza nucleofection system (program DN-100, solution P3). The Institutional Animal Care and Use Committees of Virginia Tech and the University of Alabama at Birmingham approved all the experimentation involving the use of mice. All the methods were performed in accordance with the approved guidelines. Murine EL4 T cells (TIB-39, ATCC) were cultured in RPMI supplemented with 10% FBS and 1% Pen-strep. EL4 transfections were performed using the Lonza 4D nucleofection system (program CM-120, solution SF). Immunoblot analysis was used to assess the expression levels of all transfected proteins. RNA purification and quantitative PCR with reverse transcription Cells were collected on day 5, 6 or 7 (dependent on experimental design) and RNA was purified using the Machery Nagel RNA purification kit. Complementary DNA was prepared using the First Strand Superscript II Synthesis System (Invitrogen). Quantitative PCR with reverse transcription (qRT–PCR) reactions were performed with the cDNA and gene-specific primers ( Supplementary Table 1 ) and SYBR green master mix (Bio-Rad). For the experiments in Figs 1 and 5a , PrimePCR custom plates (Bio-Rad) were used. All the samples were normalized to the Rps18 control with graphs representing data normalized to the indicated comparison condition. siRNA experiments For the siRNA experiments, both control and Prdm1 -specific siRNAs were obtained from Dharmacon (D-001210-01-20, D-043069; sequences in Supplementary Table 2 ). Primary T H 1 cells were transfected with the indicated siRNAs on day 5. Following nucleofection with siRNA, primary cells were allowed to recover in high IL-2 conditions for 24 h before gene expression analysis. Efficiency of knockdown was determined by qRT–PCR and immunoblot analysis for Prdm1 transcript and Blimp-1 protein expression, respectively. Immunoblot analysis An equal number of cells were collected and subjected to immunoblot analysis to determine protein expression levels of Bcl-6 (BD Biosciences, 561520, dilution 1:500), Blimp-1 (Genscript, A01647, dilution 1:500), STAT5 (Santa Cruz, sc-835, dilution 1:5,000), phospho-STAT5 (pY694, BD Biosciences, 611964, dilution 1:5,000) and V5-tagged proteins (Invitrogen, R960-25, dilution 1:5,000). In brief, separation of lysates by SDS–polyacrylamide gel electrophoresis was followed by immunoblot analysis. GAPDH (Santa Cruz, sc-25778, dilution 1:2,500) or β-actin (Genscript, A00730, dilution 1:10,000) expression was monitored to ensure equal protein loading. Additional information for antibodies can be found in Supplementary Table 3 and uncropped versions of all immunoblots are provided in Supplementary Fig. 5 . ChIP assay The ChIP assay was performed as published [12] . In brief, chromatin was harvested from T FH /T CM -like cells treated with and without IL-7 as indicated. Chromatin was incubated with antibodies to either STAT5 (Santa Cruz, sc-835x, 5 μg per IP) or IgG (Abcam, ab6709, 5 μg per IP) control and the precipitated DNA was analysed by qPCR with gene-specific primers ( Supplementary Table 1 ). Samples were normalized to a standardized total input DNA control followed by subtraction of the IgG antibody as a control for the nonspecific background. The final value represents the percent enrichment of STAT5-specific signal. Promoter–reporter analysis S ell (−1,755 to +79 bp), Ccr7 (−1,470 to +113 bp) and Tbx21 (−1,893 to +194 bp) promoter–reporter vectors were prepared by cloning regulatory regions of each gene into the pGL3-basic luciferase reporter construct (Promega). EL4 cells were co-transfected with the promoter–reporter constructs in combination with the indicated expression vectors as well as a TK- renilla control plasmid (Promega) to normalize for transfection efficiency. Transfections were harvested after 16–24 h and samples were analysed with the Dual-Luciferase Reporter system (Promega). Flow cytometry Fluorochrome-labelled α-IL-6Rα (P22272, dilution 1:10), α-IL-7R (A7R34, dilution 1:10), α-CD62L (95218, dilution 1:20), α-Cxcr5 (614641, dilution 1:10) and respective isotype control antibodies were purchased from R&D. α-Ccr7 (4B12, dilution 1:50), α-IL-2Rα (PC61.5, dilution 1:50), α-IL-7R (SB/199, dilution 1:10) and α-CD62L (MEL-14, dilution 1:100) were purchased from eBioscience. Non-viable cells were excluded using e520 or e450 viability dye (eBioscience), Sytox Green or Blue (Life Technologies) or propidium iodide (BD Biosciences). For the staining procedure, cells were collected on day 6 (3 days post transition to low IL-2 conditions) and subjected to labelling and sorting as indicated. Briefly, cells were pelleted, washed in 500 μl of 1 × FACS buffer (2% FBS, 1% BSA, 0.1% NaNH 3 ), and then stained with indicated fluorochrome-conjugated antibody. Following staining with fluorochrome-conjugated antibodies and viability dye, cells were washed three times in 1 × FACS buffer and then resuspended for analysis on either an Accuri C6 flow cytometer or Sony SH800. All the obtained data were analysed using FlowJo Software. Cell sorting and droplet digital PCR Day 6 IL-6Rα + /IL-7R + DP cells were sorted ( ∼ 500,000 cells) using a Sony SH800 using a 100 μm chip under purity-sort mode and cDNA was prepared as described above (see qRT–PCR). Droplet Digital PCR reactions were performed using gene-specific primers diluted in 2 × master mix (Qx200 ddPCR EvaGreen Supermix, Bio-Rad). Droplets were generated using a Bio-Rad Automated Droplet Generator and end-point PCR was performed. Droplets were then read using a Qx200 Digital PCR Reader using QuantaSoft Software (Bio-Rad). All the primers were diluted to optimize signal-to-noise and thresholds were set using non-template control wells. Absolute counts were normalized to Rps18 and then fold change was determined. Influenza virus infections and in vivo analysis Influenza virus infections were performed intranasally with 6,500 VFU of A/PR8/34 (PR8) in 100 μl of PBS. Cell suspensions from mLNs were prepared by passing tissues through nylon mesh. Cells from mLNs were resuspended in 150 mM NH 4 Cl, 10 mM KHCO 3 and 0.1 mM EDTA for 5 min to lyse red cells. Cell suspensions were then filtered through a 70 μm nylon cell strainer (BD Biosciences), washed and resuspended in PBS with 5% donor calf serum and 10 μg ml −1 FcBlock (2.4G2 -BioXCell) for 10 min on ice before staining with fluorochrome-conjugated antibodies or tetramer reagents. Fluorochrome-labelled α-PD-1 (J43, dilution 1:100), α-IL-7R (A7R34, dilution 1:100) and α-IL-6Rα (D7725A7, dilution 1:100) were from eBioscience. Fluorochrome-labelled α-Bcl-6 (K112.91, dilution 1:50), α-Cxcr5 (2G-8, dilution 1:50) and α-CD4 (RM4-5, dilution 1:200) were from BD Biosciences. The IA b NP 311-325 MHC class II tetramer was obtained from the NIH Tetramer Core Facility and used at a 1:100 dilution. Intracellular staining for Bcl-6 was performed using the mouse regulatory T-cell staining kit (eBioscience) following the manufacturer’s instructions. Flow cytometry was performed using a FACSCanto II (BD Biosciences) and analysed in FlowJo. Statistics All the data represent at least three independent experiments with the number of biological replicates indicated in the figure legend. Error bars represent the s.e.m. or s.d. as indicated. For statistical analysis, an unpaired t test was performed using GraphPad Prism online software. P values <0.05 were considered statistically significant. How to cite this article: McDonald, P. W. et al . IL-7 signalling represses Bcl-6 and the T FH gene program. Nat. Commun. 7:10285 doi: 10.1038/ncomms10285 (2016).